High-performance rechargeable lithium-iodine batteries using triiodide/iodide redox couples in an aqueous cathode Development of promising battery systems is being intensified to fulfil the needs of long-driving-ranged electric vehicles. The successful candidates for new generation batteries should have higher energy densities than those of currently used batteries and reasonable rechargeability. Here we report that aqueous lithium-iodine batteries based on the triiodide/iodide redox reaction show a high battery performance. By using iodine transformed to triiodide in an aqueous iodide, an aqueous cathode involving the triiodide/iodide redox reaction in a stable potential window avoiding water electrolysis is demonstrated for lithium-iodine batteries. The high solubility of triiodide/iodide redox couples results in an energy density of ~ 0.33 kWh kg −1 , approximately twice that of lithium-ion batteries. The reversible redox reaction without the formation of resistive solid products promotes rechargeability, demonstrating 100 cycles with negligible capacity fading. A low cost, non-flammable and heavy-metal-free aqueous cathode can contribute to the feasibility of scale-up of lithium-iodine batteries for practical energy storage. Advancement in clean-energy promoting renewable, safe, cost-effective and environmentally friendly energy technology is one of the most significant scientific and engineering duties to cut pollution and global warming. In particular, development of advanced electric vehicles is one of the most critical challenges in clean-energy technology to lessen air pollution and the dependence on fossil fuels. As a result, rechargeable batteries have attracted much attention for battery-powered electric motors. According to the Battery Roadmap 2010 announced by the New Energy and Industrial Technology Development Organization in Japan, the main target for rechargeable batteries is an improvement of the energy density up to 0.5 kWh kg −1 cell (1.0 kWh l −1 cell ) by 2030 ( http://www.nedo.go.jp/library/battery_rm2010_index.html ) to enable electric vehicles to extend the driving range to a comparable level with gasoline-powered internal combustion engine vehicles ( ca . 500 km). However, achieving more than three times the energy density raised from the currently employed battery systems (<0.2 kWh kg −1 cell ) ( [1] ) is an exceptional challenge, because the current battery technology has almost reached its performance limitation. Accordingly, new battery systems using new chemistries and system configurations are needed, which are capable of achieving higher energy density than the current ones. Among the new storage systems, non-aqueous lithium-sulfur (Li-S) and lithium-oxygen (Li-O 2 ) batteries have thus far shown the most promising energy density of 0.3−0.5 kWh kg −1 ( [1] , [2] ). However, their poor cycling performance does not meet the practical battery criteria, which is mostly due to the parasitic reactions in non-aqueous electrolytes such as the internal shuttling of lithium polysulfides for Li-S batteries [2] and instability of non-aqueous electrolytes from superoxide radical [2] and at high potential [3] , [4] for Li-O 2 batteries. In addition, the insoluble insulating discharge products decrease in the electronic and ionic conductivities. The alternative to make a less problematic storage system is aqueous lithium batteries [5] , [6] , [7] , [8] . The aqueous solution has a high ionic conductivity in the presence of completely ionized substances, which leads to rapid redox reactions in electrochemical cells. The idea has been to employ these aqueous electrolytes in a cathode, referred to as the aqueous cathode [9] , [10] , using redox couple reactions that do not deteriorate the aqueous cathode and electrically conductive current collector, as well as not leave over any solid product and precipitation residue at the aqueous cathode/current collector interface. The aqueous cathode can, therefore, offer negligible polarization and volume expansion. A promising aqueous cathode can be determined from the redox couples possessing high solubility and a suitable redox potential avoiding the electrolysis of water. The solubility is proportional to the energy density. In the diagram of redox couple solubility with respect to the standard reduction potential ( Fig. 1a ) ( [11] ), the triiodide/iodide (I 3 − /I − ) redox couple reaction shows a favourable solubility (over 8 mol l −1 ). The redox potential of the I 3 − /I − couples (0.536 V versus standard hydrogen electrode (SHE)) is also suitable to avoid water electrolysis. Therefore, in this work for the first time, we present the aqueous cathode operated by the I 3 − /I − redox couples and apply this for a lithium-iodine (Li-I 2 ) battery. The aqueous Li-I 2 battery we demonstrate is noticeably different from either the conventional all-solid-state or non-aqueous electrolyte-based Li-I 2 batteries, which have performed at extremely low discharge current rate or shown low Coulombic efficiency with the formation of a lithium iodide (LiI) layer [12] , [13] . The I 3 − /I − redox reaction in aqueous cathode is rapid and performed up 12 mA cm −2 of discharge current rate without serious potential drop. The aqueous Li-I 2 battery attains superior storage capacity (~ 98% of the theoretical capacity), Coulombic efficiency (>99.5%), and cyclic performance (>99.5% capacity retention for 100 cycles) which is, to the best of our knowledge, the best result among previous reports using new chemistries and system configurations. The energy density reaches ~ 0.33 kWh kg −1 , which is higher than that achieved in the conventional batteries. 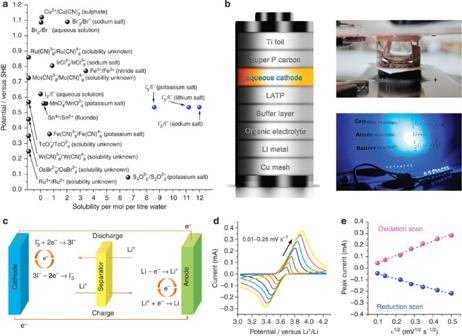Figure 1: I3−/I−redox reaction-based aqueous cathodes. (a) Diagram of the solubility of reversible redox couples in aqueous solution with respect to the standard reduction potential11. The blue balls indicate the I3−/I−redox couples with Li, Na and K salts. (b) Schematic illustration of the aqueous Li-I2battery composed of (−) Cu mesh/Li metal/organic electrolyte (1 M of LiPF6in EC/DMC)/buffer layer/ceramic separator (LATP, Li2O-Al2O3-TiO2-P2O5glass ceramic)/aqueous electrode (I2/KI)/Super P carbon/Ti foil (+) from bottom to top (left), and digital pictures of the assembled Li-I2battery (right top) and applied discharge for bulb lighting (right bottom). (c) The working concept of I3−/I−redox reaction in the aqueous Li-I2battery. (d) CV curves at sweeping rates of 0.01 (grey), 0.02 (orange), 0.05 (dark yellow), 0.08 (blue), 0.12 (cyan), 0.18 (magenta) and 0.25 (yellow) mV s−1. (e) Linearly increased oxidation (top magenta) and reduction (bottom blue) peak-currents with increasing sweeping rates (υ). Figure 1: I 3 − /I − redox reaction-based aqueous cathodes. ( a ) Diagram of the solubility of reversible redox couples in aqueous solution with respect to the standard reduction potential [11] . The blue balls indicate the I 3 − /I − redox couples with Li, Na and K salts. ( b ) Schematic illustration of the aqueous Li-I 2 battery composed of (−) Cu mesh/Li metal/organic electrolyte (1 M of LiPF 6 in EC/DMC)/buffer layer/ceramic separator (LATP, Li 2 O-Al 2 O 3 -TiO 2 -P 2 O 5 glass ceramic)/aqueous electrode (I 2 /KI)/Super P carbon/Ti foil (+) from bottom to top (left), and digital pictures of the assembled Li-I 2 battery (right top) and applied discharge for bulb lighting (right bottom). ( c ) The working concept of I 3 − /I − redox reaction in the aqueous Li-I 2 battery. ( d ) CV curves at sweeping rates of 0.01 (grey), 0.02 (orange), 0.05 (dark yellow), 0.08 (blue), 0.12 (cyan), 0.18 (magenta) and 0.25 (yellow) mV s −1 . ( e ) Linearly increased oxidation (top magenta) and reduction (bottom blue) peak-currents with increasing sweeping rates ( υ ). Full size image I 3 − /I − redox reaction in aqueous cathode of Li-I 2 batteries The I 3 − /I − redox reaction ideally occurs at 0.536 V versus SHE ( Fig. 1a ) via two-electron transfer like the following electrochemical equation (1). By using an aqueous half-cell of 1 M of KI solution, the formation of I 3 − (brown) by the oxidation of I − (transparent) and its reverse reaction could be confirmed via the colour change of electrolyte on a glassy carbon (GC) electrode (see Methods and Supplementary Fig. S1 ), which occurred around 0.57 and 0.49 V versus SHE. The I 3 − /I − redox-couple-based aqueous cathode was prepared with 1 M of aqueous KI by the addition of I 2 to adjust the I 3 − concentration. The solubility of I 2 is reasonably high in the presence of alkaline iodide, which predominantly transforms I 2 to I 3 − according to the following chemical equation (2) ( [14] ) where K is the equilibrium constant. From this, it is estimated that there is ~ 0.1 M of I 3 − in the given mixture of 0.1 M of I 2 and 1 M of aqueous KI. The potential of I 3 − /I − redox reaction can be calculated by Nernst equation (3): where E is the redox reaction potential, E o is the standard cell potential, R is the gas constant, T is the absolute temperature, n is the number of moles of electrons transferred, F is the Faraday constant, and and are the activity of I 3 − and I − , respectively. Assuming that the activity of I 3 − and I − equals to its concentration, respectively, the redox reaction potential becomes 0.508 V versus SHE in 0.1 M of I 2 and 1 M of aqueous KI. The I 3 − /I − aqueous cathode was directly used for the aqueous Li-I 2 battery. The aqueous Li-I 2 batteries consist of Li anode (Cu mesh/Li metal/organic electrolyte/buffer layer), ceramic separator, aqueous cathode, and current collector (Super P carbon/Ti foil) as shown in Fig. 1b . Li metal with 1 M of LiPF 6 in ethylene carbonate (EC)/dimethyl carbonate (DMC) electrolyte was used for the anode. The Super P carbon-coated Ti foil was employed as the current collector in the aqueous cathode. The water-stable and Li ion conductive Li 2 O-Al 2 O 3 -TiO 2 -P 2 O 5 (LATP) glass ceramic (see Supplementary Fig. S2 for the X-ray diffraction (XRD) pattern) separated the two electrodes and allowed only the Li ion to transfer across it [15] . The aqueous Li-I 2 battery is operated as follows ( Fig. 1c ). Li anode: Aqueous cathode: Total cell reaction: Cyclic voltammetry (CV) curves of the aqueous Li-I 2 battery in Fig. 1d show 3.57 V and 3.68 V versus Li + /Li for the reduction and oxidation peaks, respectively, at 0.01 mV s −1 sweeping rate and the potential difference between the reduction and oxidation peaks increased in higher sweeping rates. The linearly increased oxidation and reduction peak-currents correlated with the square root of the sweeping rate ( υ ) as shown in Fig. 1e revealed that the I 3 − /I − redox reaction was diffusion-controlled in the Li-I 2 battery [16] . The galvanostatic measurements of the prototype Li-I 2 battery showed ~ 80% Coulombic efficiency at 298 K on the first cycle of charge/discharge ( Supplementary Fig. S3a ). The deficient charge capacity was due to the low Li ion concentration (roughly 0.2 M) obtained in the aqueous cathode as the counter ion of I − , transformed from I 3 − on discharge (2Li+I 3 − →2Li + +3I − ). The limited number of Li ions could not provide sufficient ionic conductivity to balance the number of charges during the charge/discharge process and eventually terminated the charge process at the 80% point of discharge capacity (see Methods and Supplementary Fig. S4 for more details). This problem, however, could be solved simply by the addition of Li salt in the aqueous cathode. Supplementary Fig. S3b shows ~ 99.7% Coulombic efficiency for the initial cycle using 0.03 M of LiI in the presence of 0.08 M of I 2 and 1 M of aqueous KI cathode. It was also in according with ~ 99.7% Coulombic efficiency from the prototype Li-I 2 battery without LiI additive on the second cycle ( Supplementary Fig. S3a ), in which the residual Li ions stranded in the aqueous cathode after the first charge improved the ionic conductivity of Li ion during the second charge process. This ideal Coulombic efficiency is conspicuously distinguished from Li-S and Li-O 2 batteries suffering from overcharge [17] , [18] and deficient Coulombic efficiency [19] , respectively. Electrochemical performance of aqueous Li-I 2 batteries The tailored Li-I 2 batteries showed high energy density and excellent recharge ability. 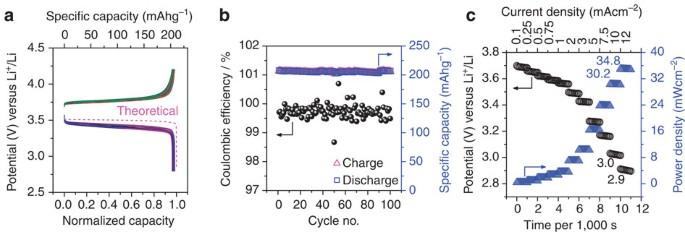Figure 2: Electrochemical performance of aqueous Li-I2batteries. (a) Hundred-times cycled charge/discharge profile at a current rate of 2.5 mA cm−2using 0.08 M of I2in the presence of 1 M of KI and 0.03 M of LiI. The magenta dashed curve indicates the theoretical discharge profile. (b) Cyclic performance presenting Coulombic efficiency and specific capacity upon charge/discharge cycles. (c) Polarization graph presenting discharge potential (black circle) and corresponding power density (blue triangle) at current rates ranging from 0.1 to 12 mA cm−2in 1 M of I2and 2 M of KI. Figure 2a presents charge/discharge curves for 100 cycles using 0.08 M of I 2 in 1 M KI and 0.03 M LiI. The specific capacity was ~ 207 mAh g −1 at a current rate of 2.5 mA cm −2 , which approaches ca . 98% of the theoretical capacity (211 mAh g −1 , the magenta line in Fig. 2a ). The energy density turned out to be ~ 0.35 kWh kg −1 calculated from the mass of aqueous cathode containing saturated I 2 and KI and Li metal in anode (see Methods) and ~ 0.33 kWh kg −1 estimated from the experimental result in I 2 saturated Li-I 2 battery ( Supplementary Fig. S5 ), which is several times higher than previously reported for alkaline aqueous cathodes [9] , [10] , [20] , redox-flow battery systems [21] and other secondary batteries based on aqueous electrolyte [5] , [6] , [22] . Furthermore, no significant capacity fading was observed during cycles. Figure 2b exhibits ~ 99.6% capacity retention and 99.5−100% Coulombic efficiency for 100 cycles, which is superior to Li-S and Li-O 2 batteries [2] , as well as other aqueous Li batteries using a solid Ni(OH) 2 cathode (95−96% for 50 cycles) [22] , and aqueous cathodes comprises Fe 3+ /Fe 2+ redox reaction [9] and Fe(CN) 6 3− /Fe(CN) 6 4− (~ 98.6%) ( [10] ). The high capacity retention also sustained in high concentration, 1 M of I 2 in the presence of 1 M KI, with ~ 100% Coulombic efficiency for 20 cycles ( Supplementary Fig. S6 ). The open circuit potential was ~ 3.8 V versus Li + /Li and the discharge and charge potentials were stable at 3.50 and 3.70 V versus Li + /Li on cycling, which resulted in overpotentials of 0.04 and 0.16 V, respectively, from the thermodynamically reversible potential of I 3 − /I − in the aqueous cathode (3.54 V versus Li + /Li). A larger overpotential on charge is due to the low ionic conductivity of LATP at a high current rate of 2.5 mA cm −2 . Nevertheless, the overpotential value at such a high current rate is still comparable to Li ion batteries [23] , [24] , and superior to Li-S ( [18] ) and Li-O 2 ( [19] , [25] , [26] ) batteries at current rates even an order of magnitude lower, demonstrating ~ 90% overall energy efficiency on cycling as shown in Supplementary Fig. S7 . Figure 2: Electrochemical performance of aqueous Li-I 2 batteries. ( a ) Hundred-times cycled charge/discharge profile at a current rate of 2.5 mA cm −2 using 0.08 M of I 2 in the presence of 1 M of KI and 0.03 M of LiI. The magenta dashed curve indicates the theoretical discharge profile. ( b ) Cyclic performance presenting Coulombic efficiency and specific capacity upon charge/discharge cycles. ( c ) Polarization graph presenting discharge potential (black circle) and corresponding power density (blue triangle) at current rates ranging from 0.1 to 12 mA cm −2 in 1 M of I 2 and 2 M of KI. Full size image Figure 2c shows a polarization graph recorded in the 0.1−12 mA cm −2 range of current rates using 1 M of I 2 and 2 M of KI. The linear reduction in discharge potential with increasing current rate ( Supplementary Fig. S8 ) arose from the larger internal resistance of the Li-I 2 battery. The power density correlated with the potential turned out to be ~ 30 mW cm −2 at 10 mA cm −2 current rate, which was more than three times higher than the first aqueous cathode [10] of Fe(CN) 6 3− /Fe(CN) 6 4− , and twice that of its flow-through-mode system [20] . More importantly, the aqueous Li-I 2 battery did not present any significant potential drop up to a current rate of 12 mA cm −2 , even though slightly unsettled discharge potentials were observed over 5 mA cm −2 , which was notably different from the previous alkaline aqueous cathodes exhibiting a greater potential drop due to the mass transport loss over 2.5 mA cm −2 of current rate [10] , [20] . It was due to the fact that the suitable reduction potential of I 3 − /I − suppresses a pronounced potential drop approaching to the electrolysis potential of water, which would otherwise cause deterioration of the battery at high current rate. The power density eventually approached ~ 34.8 mW cm −2 at 12 mA cm −2 associated with a discharge potential of ~ 2.9 V versus Li + /Li. We demonstrated reliable battery performance with high energy density on cycles in aqueous Li-I 2 battery. It was attributed to a stable working potential window. The main redox reaction occurred in the potential region of 3.5–3.7 V versus Li + /Li that was converted to 0.46–0.66 V versus SHE. Although the potential drop/increase has been shown in the potential window of 2.8–4.2 V versus Li + /Li (−0.24 to +1.16 V versus SHE) at the end of charge/discharge process the aqueous cathode containing the excessive ionic concentration was electrochemically stable [27] evidenced by neither H 2 nor O 2 evolution. The ceramic separator of LATP, current collector and aqueous cathode were stable at this operating condition. There was no significant structure and phase change of LATP on both sides communicating with the organic (EC/DMC with Li salt in the anode side) and aqueous (I 2 /KI/LiI in the cathode side) electrolytes, confirmed by identical XRD patterns before ( Supplementary Fig. S2 ) and after 100 cycles ( Fig. 3a ). Nyquist plot using electrochemical impedance spectroscopy also revealed negligible decrease in ionic resistance after 100 cycles ( Supplementary Fig. S9 ). The sturdy LATP ceramic separator performed Li ion commute between anode and cathode on cycling. Inductively coupled plasma optical emission spectrometry exhibited almost similar Li ion concentration in the fresh (27.7 mM) and 100-cycled (27.1 mM) aqueous electrodes ( Fig. 3b ). In addition, the current collector of Super P carbon/Ti did not deteriorate on cycling. We could not find any corrosion evidence of Ti foil by naked eye. Scanning electron microscopy images in Fig. 3c and corresponding energy dispersive spectrometer analysis using transmission electron microscopy in Supplementary Fig. S10 revealed neither morphological change nor a precipitation layer on the Super P carbon. It was evident that the aqueous cathode was capable of sustaining over 100 cycles with the LATP separator and current collector. Indeed, the aqueous Li-I 2 battery constructed with the aqueous cathode collected from the 100-cycled battery displayed comparable performance to the fresh one. This rebuilt battery delivered a capacity of ~ 200 mAh g −1 ( Fig. 3e ) and >99.5% Coulombic efficiency for 50 cycles without any significant capacity fading ( Fig. 3f ). 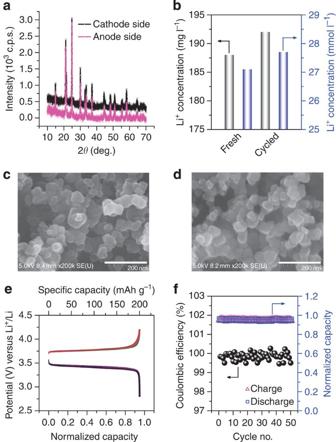Figure 3: Analyses of 100-times cycled aqueous Li-I2batteries and their post electrochemical performance. (a) XRD patterns of LATP communicating with anode (magenta) and cathode (black) electrolytes for 100 cycles. (b) Inductively coupled plasma optical emission spectrometry analysis of Li ion concentration. The Li ion concentration was 188 and 192 mg l−1(black column) or 27.1 and 27.7 mM (blue column) for the fresh and 100-cycled aqueous electrodes, respectively. Scanning electron microscopy images of Super P carbon before (c) and after (d) 100 cycles. Scale bars, 200 nm. Charge/discharge profile (e) and cyclic performance (f) upon 50 cycles from the battery constructed from 100-cycled aqueous electrode (I2/KI/LiI with 0.08/1/0.03 M). Figure 3: Analyses of 100-times cycled aqueous Li-I 2 batteries and their post electrochemical performance. ( a ) XRD patterns of LATP communicating with anode (magenta) and cathode (black) electrolytes for 100 cycles. ( b ) Inductively coupled plasma optical emission spectrometry analysis of Li ion concentration. The Li ion concentration was 188 and 192 mg l −1 (black column) or 27.1 and 27.7 mM (blue column) for the fresh and 100-cycled aqueous electrodes, respectively. Scanning electron microscopy images of Super P carbon before ( c ) and after ( d ) 100 cycles. Scale bars, 200 nm. Charge/discharge profile ( e ) and cyclic performance ( f ) upon 50 cycles from the battery constructed from 100-cycled aqueous electrode (I 2 /KI/LiI with 0.08/1/0.03 M). Full size image By using the I 3 − /I − redox couples, the aqueous Li-I 2 battery has several advantages to achieve a reliable clean-energy storage system. The I 2 /KI aqueous electrolyte provides near-neutral pH (~ 6.3 in the as-prepared electrolyte, ~ 7.2 in both I 2 and KI the saturated electrolyte), which removes the concern for degradation of the ceramic separator [10] and additional chemical treatment to facilitate redox reactions on the working system [9] . The aqueous KI enables the aqueous Li-I 2 battery to be scaled up with a low cost by eliminating the costly organic electrolyte and Li salts in the cathode. Besides, I 2 /KI electrolyte is non-flammable and heavy-metal free. In addition, again, the aqueous cathode containing the I 3 − /I − redox couples does not leave any solid product, which leads to no volume expansion and promotes adequate recharge ability. The redox reaction potential is also suitable for use in aqueous solution, thereby rendering no deterioration of the battery at high current rate despite the cooperation with low ionic conductivity of LATP ceramic separator. Therefore, the aqueous cathode using the I 3 − /I − redox couples shows great promise to constitute the new generation of energy storage system to satisfy both high energy density and low environmental impact, and could be suitably scaled up subsequent to development of a ceramic separator with higher mechanical strength. In summary, the I 3 − /I − redox reaction-operated aqueous Li-I 2 battery exhibited excellent cyclic performance with considerable energy and power densities. Ideal Coulombic efficiency and capacity retention with no degradation of cathode establish the aqueous Li-I 2 battery as one of the outstanding post Li batteries. The specific energy density (~ 0.33 kWh kg −1 ) is fairly promising in comparison to the conventional lead-acid, nickel-metal hydride and Li ion batteries, and can be further improved to be ~ 0.4 kWh kg −1 using NaI or LiI instead of aqueous KI as referred to the solubility diagram in Fig. 1a . The aqueous cathode system can be also extendable to aqueous Na-I 2 and K-I 2 batteries. We believe that this energy storage system can be scaled up with a reasonably increased energy density by combining a flow-through-mode system. Preparation of aqueous Li-I 2 batteries The preparation and assembly of the anode side were conducted in an Ar-filled glove box (<1 p.p.m. of H 2 O and O 2 , Kiyon). A thin and flat Li metal (Honjo) attached to a copper (Cu) mesh (Nilaco Corporation, 100 mesh) was set on a cylindrical glass shell. A polymer buffer layer (Celgard 2500, received from Celgard) was inserted between the Li metal and LATP to impede the formation of a highly resistive precipitation layer from the ceramic separator [28] . An organic electrolyte of 1 M LiPF 6 (Aldrich) in ethylene carbonate (EC, Kishida Chemicals)/dimethyl carbonate (DMC, Kishida Chemicals) with volume ratio 3:7 was added into this glass cylinder. LATP (Li 2 O-Al 2 O 3 -TiO 2 -P 2 O 5 ) glass ceramic separator (Ohara Corporation, ~ 180±20 μm in thickness) was fixed on top of the glass cylinder thus sealing in the anode. To prepare the current collector and aqueous cathode, Super P carbon (received from Timcal) and a polyvinylidene fluoride binder (PVDF, received from Kynar) were mixed with in an 80:20 mass ratio in N -methyl-2-pyrrolidone. This carbon slurry was cast on a titanium (Ti) foil (99.5% of purity, Nilaco Corporation, 40 μm in thickness) with a loading density of 1 mg cm −2 carbon and dried at 115 °C for 12 h in air to remove any residual solvent. The current collector of Super P carbon-loaded Ti foil was stuck on the other cylindrical shape of the glass shell, in which the aqueous cathode containing I 2 (99%, Wako Chemicals), KI (99.5%, Wako Chemicals), and LiI (99.9%, Wako Chemicals) was added with a total volume of 150 μl, which was then sealed with the backside of the LATP employed in the anode assembly. The completed battery had a configuration of (−) Cu mesh/Li metal/organic electrolyte/buffer layer/LATP/aqueous cathode/Super P carbon/Ti foil (+) ( Fig. 1b ). The geometric areas of the current collector and the ceramic separator were ~ 0.2 cm 2 (5 mm in diameter) and 0.5 cm 2 (8 mm in diameter), respectively. Electrochemical measurements The I 3 − /I − electrochemical reaction was investigated using a potentiostatic method of CV and a galvanostatic method of charge/discharge curve at room temperature in 1 atm using a battery cycler (WBCS3000, WonATech). The CV curves of the aqueous Li-I 2 batteries were recorded at sweeping rates from 0.01 to 0.25 mV s −1 in the potential range from 3.04 to 4.24 V versus Li + /Li. The battery performance was carried out at 2.8 and 4.2 V versus Li + /Li for the cutoff discharge and charge potential, respectively. The current rate estimated from the applied current with the geometrical area of current collector was from 0.1 to 12 mA cm −2 . The capacity was calculated from the mass of active species of I 2 , for example, ca. 3 mg from 0.08 M of I 2 in 150 μl of total aqueous cathode. I 3 − /I − redox reaction The I 3 − /I − redox reaction was investigated via potentiostatic mode (VMP3, Biologic). The CV was examined in a half-cell of 1 M KI at a sweeping rate of 10 mV s −1 . A polished GC was used as the working electrode with a Pt wire as the counter electrode, and a saturated calomel electrode as the reference electrode. Supplementary Fig. S1 shows the optical images of GC electrode surface in 1 M aqueous KI and with the corresponding CV curve. From open circuit potential (OCP, ~ 0.12 V), the curve was swept from (1) negative (black), (2)—(3) positive (blue) and (4)—(5) negative (black) potential direction in the potential range from 0.1 to 0.8 V. The oxidation reaction (3I − →I 3 − +2 e − ) was observed from ~ 0.32 V by the CV curve and the electrolyte colour on the GC surface changed from transparent (I − ) to brown (I 3 − ). The I 3 − formed during (3)—(4) sweeping diffused out from the GC surface. Disappearance of I 3 − close to the GC surface could be observed at ~ 0.25 V due to the reduction reaction (I 3 − +2 e − →3I − ). The reduction and oxidation reactions, therefore, occurred ~ 0.494 and ~ 0.564 V versus SHE, presenting somewhat the resistive behaviour from the thermodynamically reversible potential (0.536 V versus SHE). Diffusion-controlled behaviour in aqueous Li-I 2 batteries Supplementary Fig. S4 shows quantitatively simulated diffusion-controlled charge/discharge behaviour of the prototype Li-I 2 battery (the first cycle of Supplementary Fig. S3a ) in terms of the ionic conductivities of LATP ( σ (LATP), 10 −3 −10 −4 S cm −1 ) ( http://www.ohara-inc.co.jp/en/product/electronics/licgc.html#04 ), Li ion ( σ (Li + )) ( [29] ), I − ( σ (I − )) ( [29] ), I 3 − ( σ (I 3 − )) ( [30] ), organic electrolyte ( σ (organic) from 1 M LiPF 6 in EC/DMC in the anode side, ≈1.1 × 10 −2 S cm −1 ) ( [31] ) and the applied current rate ( σ ( J )). The σ ( J ) (olive solid line) at a current density of 2.5 mA cm −2 was estimated from the charge/discharge profile in Supplementary Fig. S3a according to equations (equations 7 and 8): Discharge: Charge: where J was the current rate (2.5 mA cm −2 ), l was the distance between anode and cathode (3 mm), E discharge was the discharge potential, E charge was the charge potential, and E o , R , T , n , F , and are identical to Nernst equation (equation 3). The σ (organic) (black dashed line) and σ (I − ) (white solid line) were a few orders of magnitude higher than the others due to the high concentration and thus were not involved in the termination of discharge and charge process. The typical σ (LATP) (blue dashed line) obtained from Li ion diffusion in the LATP was higher than σ ( J ) on discharge, which contributed to smooth mass transport of Li ions from the anode to the aqueous cathode. The discharge capacity was predominantly governed by the I 3 − concentration through the I 3 − /I − redox reaction ( ). The σ (I 3 − ) (pink solid line) steeply decreased at the end of discharge and eventually reached σ ( J ) as marked by the black square. The normalized discharge capacity was ~ 0.97, which was consistent with the experimentally obtained capacity of ~ 0.98 (normalized). Upon charge, abundant I − ions ( σ (I − )) in aqueous KI did not contribute to the termination of the charge process. Instead, σ (Li + ) (orange solid line) determined the termination by closely reaching σ ( J ). The limited Li ion concentration (roughly 0.2 M) in the aqueous cathode as the counter ion of I − transformed from I 3 − could not provide sufficient ionic conductivity to retain the charge process up to the same capacity of discharge. It was also probably related to the high resistance of LATP to migration of Li ions from the aqueous cathode to the anode. The normalized capacity of ~ 0.79 was deduced as indicated by the black square, which was comparable to the experimentally obtained value of ~ 0.80 (normalized). With regard to the diagram shown in Supplementary Fig. S4 , several methods can be proposed to increase Coulombic efficiency. The first one is to increase the concentration of Li ion or I 2 in the aqueous electrode, which can increase the σ (Li + ) and retain the charge process further. The second is to decrease the applied current rate ( J ) during charge. Optimized electrode design such as shortening the I 3 − or Li ion diffusion distance ( l ) would also be beneficial. Among them, the addition of Li salt in the aqueous cathode is the simplest route to increase the Coulombic efficiency while maintaining the existing battery performance. It is evidenced by ~ 100% Coulombic efficiency on the second cycled battery ( Supplementary Fig. S3a ), in which the residual Li ions stranded in the aqueous cathode after the first charge increased Li ion conductivity. The additional Li salt in the fresh aqueous cathode improved Coulombic efficiency at the initial cycle. Supplementary Fig. S3b shows ~ 99.7% Coulombic efficiency by adding 0.03 M of LiI in the presence of 0.08 M of I 2 and 1 M of KI. Estimation of energy density Energy density of the aqueous Li-I 2 battery based on the total weight of the aqueous cathode and Li metal anode can be estimated from equation (9): where ED is the energy density (kWh kg −1 ), E rev (V) is the reversible potential (3.576 V versus Li + /Li), Q is the theoretical capacity of I 2 (211 Ah kg −1 ), and M anode+cathode (kg) is the total mass of Li metal anode ( m Li ) and aqueous cathode, which is itself the sum of the mass of I 2 ( m I 2 ), alkali iodide ( m XI, X=K, Li or Na ) and water ( m H 2 O ). Considering the high solubility (~ 8.5 mol l −1 ) of I 3 − /I − ( Fig. 1a ) and I 2 in aqueous KI (equation 2), m I 2 , m XI and m Li is 2.16, 1.41 and 0.118 kg, respectively, in the given 1 kg of aqueous solution ( mml_m H 2 O ) at 298 K. The specific energy density values were thus estimated to be 0.35 kWh kg −1 or 0.70 kWh l −1 (mass density at 298 K: ~ 2 kg l −1 ). The estimated value is consistent with the experimental result of 0.33 kWh kg −1 ( Supplementary Fig. S5 ). When using LiI or NaI instead of KI, m I 2 , m XI and m Li were 2.84, 1.50 and 0.16 kg for LiI, and 3.05, 1.80 and 0.17 kg for NaI, respectively. The specific energy density values were thus estimated to be 0.39 kWh kg −1 for LiI and 0.38 kWh kg −1 for NaI, respectively. Characterizations XRD patterns were attained from a parallel beam XRD instrument (Smartlab, λ CuKα =1.542 Å, Rigaku). Inductively coupled plasma optical emission spectrometry characterization was performed on a Varian 720-ES. Scanning electron microscopy observation was performed on a Hitachi S-4800T. Transmission electron microscopy and energy dispersive spectrometer analysis was performed on a JEOL JEM-2100F. How to cite this article: Zhao, Y. et al . High-performance rechargeable lithium-iodine batteries using triiodide/iodide redox couples in an aqueous cathode. Nat. Commun. 4:1896 doi: 10.1038/ncomms2907 (2013).